Higher levels of multiple ecosystem services are found in forests with more tree species Forests are of major importance to human society, contributing several crucial ecosystem services. Biodiversity is suggested to positively influence multiple services but evidence from natural systems at scales relevant to management is scarce. Here, across a scale of 400,000 km 2 , we report that tree species richness in production forests shows positive to positively hump-shaped relationships with multiple ecosystem services. These include production of tree biomass, soil carbon storage, berry production and game production potential. For example, biomass production was approximately 50% greater with five than with one tree species. In addition, we show positive relationships between tree species richness and proxies for other biodiversity components. Importantly, no single tree species was able to promote all services, and some services were negatively correlated to each other. Management of production forests will therefore benefit from considering multiple tree species to sustain the full range of benefits that the society obtains from forests. Ecosystems provide a wealth of benefits to human society, and the provision of such ecosystem services depends fundamentally on functions performed by organisms [1] . This has led scientists to enquire how the diversity and composition of communities may regulate ecosystem functions [2] , [3] . A large body of evidence has established that species diversity promotes ecosystem functions under experimental conditions [4] , [5] . There are, however, many exceptions to the positive diversity–function relationship [6] . In addition, most experiments have been conducted at limited temporal or spatial scales (but see refs 7 , 8 ). It is thus uncertain if conclusions based on results from these studies can be extended to the scales relevant to policy makers. Thus far, studies that manipulated biodiversity and monitored the consequences mainly focused on ecosystem functions, but because functions have complex links to ecosystem services [1] , [9] , the policy implications of these studies are unclear [5] . There are relatively few large-scale observational studies explicitly aimed at quantifying the importance of biodiversity, and these have mostly analysed single-ecosystem functions or services [10] , [11] , [12] . Furthermore, while there are multiple functions that regulate services from ecosystems, few studies have investigated the role of biodiversity for multiple ecosystem functions jointly (but see, refs 13 , 14 , 15 , 16 ), and none of these have focused on services per se . In a recent comprehensive review, a majority of the included ecosystem services were related to biodiversity in the direction expected from predictions [3] . However, for many of the studied services, the evidence for beneficial effects of biodiversity was mixed, or there were not enough data for a thorough evaluation [3] . Studies that explicitly investigate the link between biodiversity and multiple ecosystem services across regional scales are thus urgently needed if research is to be informative for management and policy, such as the Intergovernmental Platform on Biodiversity and Ecosystem Services [17] . We examined the relationships between multiple ecosystem services and both tree species richness and tree biomass in boreal and temperate forest. These extensive biomes are of high global importance [1] , constituting around 27% (8.7 million km 2 ) and 16% (5.2 million km 2 ) of the world’s forests, respectively [18] . The majority of studies on the importance of tree diversity have focused on productivity, and there is evidence for both non-significant [19] and positive effects [20] . We studied production forests, that is, forests that are subjected to a silvicultural system of harvesting and planting or natural regeneration from seed trees. Production forest is the dominant system in the sampled region, which covered an area of 400,000 km 2 and a span of 13.7 degrees of latitude. These forests are relatively species poor. The maximum number of tree species in any one sampling plot in our study was 10 ( Supplementary Fig. S1 ), and only 1.5% of the plots hosted more than five species. Six ecosystem services [1] were included: tree biomass production, topsoil carbon storage, berry production, game production potential, understory plant species richness and dead wood occurrence. Production of tree biomass is a major global industry, contributing about US$ 400 billion to the annual gross world product in terms of wood [1] . Forests and their soils store about 45% of the terrestrial carbon, and act as a crucial sink for anthropogenic carbon emissions [21] . Both production of berries and game are of large monetary and recreational value in many countries [1] . Dead wood occurrence represents a supporting function for other ecosystem services, as it affects ecological processes such as nutrient cycling and soil formation [1] , [22] , and it also indicates several other components of biodiversity. Understory plant species richness differs somewhat from the other five ecosystem services, as it is not linked to biological processes or biological production, but instead can be classified as a cultural ecosystem service that provides aesthetic, educational and recreational value to human beings [1] . Alternatively, and with recent terminology, understory plant species richness may be viewed as having a value of its own [23] . Safeguarding biodiversity at all levels of organization is also a central goal of the Convention on Biological Diversity. Relationships between tree species richness and the services The relationships between tree species richness and tree biomass production, berry production (of bilberries) and game production potential were positively hump-shaped ( Fig. 1a ), taking into account important environmental variables, such as climate, soil nutrients and forest age ( Methods ). On average, biomass production at the mean forest age was 54% greater with five tree species than with only one species ( Fig. 1a ). Corresponding percentages for berry production and game production potential were 45% and 20%, respectively. Soil carbon storage and understory plant species richness increased with tree species richness ( Fig. 1b ). Soil carbon storage was 11% greater, and understory plant species richness 31% greater, with five than with one tree species. The occurrence of dead wood increased at high tree species richness ( Fig. 1f ). An alternative way of evaluating how productivity changes with tree species richness is to quantify the probability that a given species richness would have higher productivity than a monoculture. In our analyses, tree biomass production is 41% more likely to be higher on plots with five species than on plots with one species ( Supplementary Fig. S2 for details, additional statistics and corresponding percentages for the other five services). Excluding the effect of the biomass of individual tree species from the models did not change the positive relationships between the services and tree species ( Supplementary Fig. S3 ). 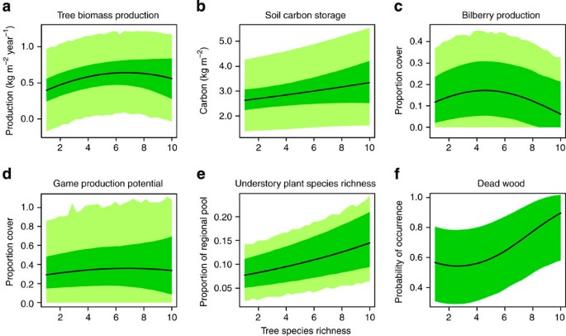Figure 1: Relationships between tree species richness and ecosystem services. (a) Tree biomass production; (b) soil carbon storage; (c) bilberry production; (d) game production potential; (e) understory plant species richness; (f) occurrence of dead wood. We show mean relationships (black) and 95% Bayesian confidence intervals for the relationships excluding (dark green) and including the residual variation (light green). Other model explanatory variables were kept at mean levels. Figure 1: Relationships between tree species richness and ecosystem services. ( a ) Tree biomass production; ( b ) soil carbon storage; ( c ) bilberry production; ( d ) game production potential; ( e ) understory plant species richness; ( f ) occurrence of dead wood. We show mean relationships (black) and 95% Bayesian confidence intervals for the relationships excluding (dark green) and including the residual variation (light green). Other model explanatory variables were kept at mean levels. Full size image Individual tree species and services None of the six ecosystem services was consistently explained by the biomass of the same tree species ( Fig. 2 ). For example, there were strong positive relationships between the biomass of spruce and tree biomass production and occurrence of dead wood, while pine biomass was positively related to bilberry production, and birch biomass to soil carbon storage. Beech was not positively related to any service. 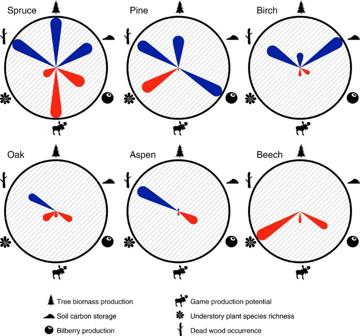Figure 2: Strength of the relationships between tree biomasses and ecosystem services. The lengths of the ‘petals’ in these flower diagrams (one diagram for each tree species) reflect transformed effect sizes for the relationships in the main models. Specifically, the effect sizes (βnin equation (1)) have been transformed to range between 0 and 1, so that for each ecosystem service the effect size for the tree species with the greatest effect equals the absolute value of 1. Blue are positive relationships, red are negative relationships, and the outer circles represent the maximum value of |1|. The six ecosystem services are labelled by their respective symbols. Figure 2: Strength of the relationships between tree biomasses and ecosystem services. The lengths of the ‘petals’ in these flower diagrams (one diagram for each tree species) reflect transformed effect sizes for the relationships in the main models. Specifically, the effect sizes ( β n in equation (1)) have been transformed to range between 0 and 1, so that for each ecosystem service the effect size for the tree species with the greatest effect equals the absolute value of 1. Blue are positive relationships, red are negative relationships, and the outer circles represent the maximum value of |1|. The six ecosystem services are labelled by their respective symbols. Full size image Relationships between ecosystem services Some of the services were positively related to each other ( Fig. 3 ), but we also found some notable trade-offs. First, there were trade-offs between tree biomass production and occurrence of dead wood, game production potential and bilberry production. Second, dead wood occurrence and game production potential were negatively correlated. 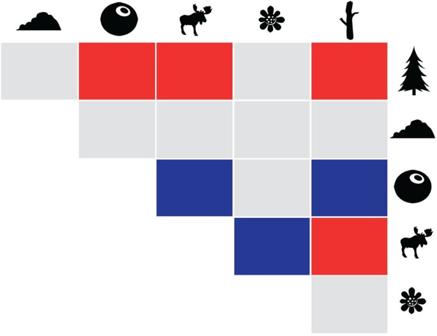Figure 3: Pairwise relationships between ecosystem services. Blue are positive and red are negative relationships. Grey reflects relationships with no established inter-relationship. The six ecosystem services are labelled by their respective symbols. Figure 3: Pairwise relationships between ecosystem services. Blue are positive and red are negative relationships. Grey reflects relationships with no established inter-relationship. The six ecosystem services are labelled by their respective symbols. Full size image The pros and cons of species mixtures for productivity and other ecosystem functions have been discussed at length since the early 19th century [2] , [24] , [25] . Not until recently, however, have scientists begun to explicitly investigate how species diversity might be important for the simultaneous provision of multiple functions or services [13] , [14] , [15] , [26] , [27] . Our results from boreal and temperate production forests show that the relationships between tree species richness and multiple ecosystem services were positive to positively hump-shaped, and that all services attained higher levels with five tree species than with one species. Although the relatively high level of tree biomass production with five compared with one tree species may seem both impressive and surprising, we note that similar effect sizes have been found previously [11] . Another observational study, in which climatic and environmental conditions were controlled for, also found a strong and positive effect of tree diversity on productivity [12] . Because controlled field studies on mixed-stand effects have revealed both non-significant and positive effects of diversity [19] , [20] , future research should aim to understand and reconcile results from controlled experiments and observational studies. There are, unfortunately, no previous studies on the relationships between tree species richness and the other five services that allow for comparisons with our findings. We found little support for a general importance of the biomass of particular species in explaining all services ( Fig. 2 ). The finding that different species were most strongly related to different services indicates that monoculture practices will lead to reduced provision of at least some of the services we considered. For example, among all tree species considered, only pine was strongly and positively related to bilberry production (see also ref. 28 ) and birch showed the strongest positive relationship with soil carbon storage. As such, our results suggest the importance of tree species mixtures for the continued provisioning of ecosystem services from the 2-billion hectares of forest in the world currently managed as production forests or used for multiple purposes (55% of all forests) [29] . The results also indicate trade-offs between some services ( Fig. 3 ). The trade-off between tree biomass production and dead wood occurrence is probably an effect of stand age; tree production generally decreases with age, whereas the opposite is true for occurrence of dead wood [30] . The negative correlation between dead wood occurrence and game production potential is most likely also partly explained by forest stand age; herbivore forage plants are more common in young forests, whereas dead wood more commonly occurs in old forests. Negative relationships between tree biomass production and the production of both bilberry and food for game are likely consequences of light limitation and lower precipitation through-fall at the ground level in closed productive forests [31] . Unlike previous findings [32] , we thus found that some ecosystem services may come at the cost of others. Identifying such trade-offs is highly relevant for policy, enabling users of forest ecosystems to understand and balance the pros and cons of different management scenarios [33] . Although the trade-offs we found imply that it will be difficult to maximize all ecosystem services simultaneously at the stand scale, the positive relationships between tree diversity and individual services ( Fig. 1 ) suggest that adjacently located monocultures would not optimize the provision of ecosystem services at the landscape scale. Instead, adjacent stands, each with multiple species but in different combinations, might be the best way to provide multiple ecosystem services at the landscape scale. The negligible effects of the biomass of single tree species on the relationship between tree species richness and ecosystem services in our study suggest complementarity among tree species, for example, resource partitioning, often referred to as ‘complementarity effects’ (or effects of species richness per se ) in experimental studies [5] . Interactions between plants and associated microbiota, and higher resistance of a diverse community to disease, insects or pathogens may also be factors explaining the observed relationships between some of the services and tree species richness [34] . Additional environmental conditions may directly or indirectly explain some of the unexplained variation in the services [34] , [35] . For example, nitrogen availability (not measured in the Swedish National Forest Inventory) may influence forest productivity. However, the ratio of total carbon to total nitrogen in the topsoil that we used is a good indicator of nitrogen availability [36] . Also, non-measured environmental variables that are correlated with altitude or latitude could be important; for example, plots in the mountain region (in northwest Sweden) generally have fewer tree species ( Supplementary Fig. S1 ). However, we accounted for temperature and humidity, which are the most important climate variables and correlated with altitude and latitude. Moreover, maximum tree species richness was relatively evenly distributed across the sampling region ( Supplementary Fig. S1 ). While our analyses were on the regional scale, there certainly may be differences at the local scale in the strength of the relationships between tree species richness and ecosystem services. All services may thus not be maximized similarly within landscapes across the whole sample region. Furthermore, we focused on the current distribution and composition of forests, but future changes in the environment may affect ecosystem services both directly and indirectly [37] . Global change may thus result in society not having all the management options currently available. Scenarios of changes in forest species composition and richness due to global change must be considered in analyses of future provisioning of ecosystem services [38] . The majority of previous efforts to disentangle the effects of tree species richness on ecosystem functions or services in forests have focused on productivity of woody biomass [11] , [12] , [39] , [40] . Mixed forest stands can indeed be more productive than monocultures [20] , and several studies have found large-scale positive relationships between tree diversity and wood production [11] , [12] , [41] . Positive relationships between biodiversity and individual ecosystem functions or services have also been observed in aquatic realms, such as the open ocean [42] , the deep sea [43] , coral reefs [44] and lakes [45] . Our study, which accounts for important environmental conditions, shows consistent positive relationships between tree species richness (contrasting plots with five and one tree species) and multiple ecosystem services. It also highlights the importance of conserving a variation of tree species, to safeguard a future potential of high levels of multiple ecosystem services. As such, our research expands on previous work [16] , [46] , none of which considers multiple services. Our study revealed complementarity among species; no single species can sustain multiple services at high levels simultaneously. This is particularly pertinent at a time when demands on ecosystems to provide humans with several important services are increasing [47] at the same time as global change and human expansion is threatening the integrity of ecosystems, their biodiversity and functioning [1] , [3] , [44] , [48] . Our results strongly support the integration of production and conservation in natural resource management, and align with the ‘ecosystem approach’, the primary framework for action under the Convention of Biodiversity [49] . We show that moving towards multi-species management can better realize the full potential of several economically, ecologically and culturally valuable ecosystem services. Description of the data We used a nationwide forest data set from the Swedish National Forest Inventory and the Swedish Survey of Forest Soils and Vegetation. The inventory uses a randomly planned regular sampling grid [50] , and includes around 4,500 permanent tracts with each tract being surveyed once every 5 years. The tracts, which are rectangular in shape and are of different dimensions in different parts of the country, consists of 8 (in the north) to 4 (in the south) circular sample plots (each plot 314 m 2 ). From the Inventory database, we extracted data from 1999 to 2002. We used only plots on ‘productive forest’ (average production of standing volume, stem volume over bark >1 m 3 ha −1 year −1 ), which had not been harvested, cleared or thinned during the previous 5 years before the survey. The previous time period of 5 years was also used for calculating biomass production. To be included in our analyses, the plots had to be located on only forest land, for example, not including any river, road, grassland and so on. We excluded plots where the biomass production of any of the focal tree species was greater than the 99% quantile (which is the standard procedure in analyses of data from the Swedish National Forest Inventory). This procedure excluded plots with unrealistically high values of production. Our selection resulted in a data set with a total of 4,335 sample plots distributed across 1,401 tracts. We included explanatory variables hypothesized to explain the variation in the six modelled ecosystem services, and squared variables and interactions, whenever biologically reasonable (see descriptions below, Fig. 4 and Supplementary Table S1 ). 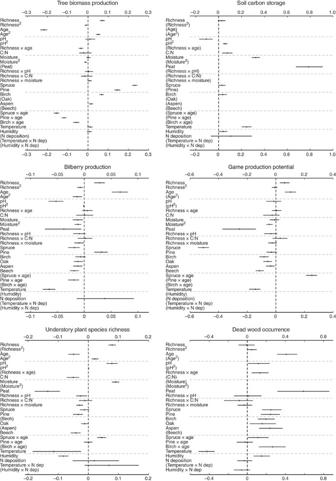Figure 4: Parameter estimates for the main model for each ecosystem service. The modes (vertical lines) and the 95% Bayesian confidence intervals (thin horizontal lines) for the parameters (βnin equation (1) andρmin equation (3)) are shown for each service (tree biomass production, soil carbon storage, bilberry production, game production potential, understory plant species richness and occurrence of dead wood). Variables or interactions in parentheses were not included in the final main model. Dashed lines are for visual aid. Figure 4: Parameter estimates for the main model for each ecosystem service. The modes (vertical lines) and the 95% Bayesian confidence intervals (thin horizontal lines) for the parameters ( β n in equation (1) and ρ m in equation (3)) are shown for each service (tree biomass production, soil carbon storage, bilberry production, game production potential, understory plant species richness and occurrence of dead wood). Variables or interactions in parentheses were not included in the final main model. Dashed lines are for visual aid. Full size image Statistical modelling To model the six ecosystem services as a function of tree species richness, we used hierarchical Bayesian-generalized linear models [51] . The Bayesian approach is convenient for fitting complex hierarchical models with a formal mathematical treatment of the natural variability and data uncertainty, for example, when the recording of the explanatory variables is incomplete. For each ecosystem service, we fitted the following models: the main model, on which our results are based unless otherwise mentioned ( Figs 1 and 2 ); a model aimed to investigate how the tree species biomasses affected the relationship between tree species richness and the services, specifically the main model but excluding the tree biomass variables ( Supplementary Fig S3 ); five models aimed to investigate the pairwise relationships between the ecosystem services, excluding all other explanatory variables ( Fig. 3 ). In the following, we exemplify the modelling using understory plant species richness as the response variable. Corresponding models were fitted for the other five ecosystem services. We assumed that the understory plant species richness followed an overdispersed Poisson distribution with mean, μ p , t ( Supplementary Table S2 ). We modelled this mean, transformed by the ln link function ( Supplementary Table S2 ), g (), on plot p =1, …, P ⩽ 8, on tract t =1, …, T ⩽ 1,394 as where, X p , t is a design matrix of n plot-level explanatory variables, β n is a vector of associated effect-size parameters, and P p , t is the regional species pool (see description of understory plant species richness). Explanatory variables were centred and standardized. As we included the log of the regional species pool, we in fact modelled the proportion of the regional species pool. The parameters ɛ p , t are overdispersion contributions, where ɛ p , t ∼ N (0, σ ), which means normally distributed with mean=0 and s.d.= σ . For normally distributed ecosystem services ( Supplementary Table S2 ), ɛ p , t are residual contributions. The tract-level ‘intercept’ parameters α t were modelled further as where σ α is the s.d., and where Z t is a design matrix of m =1, …, M ⩽ 5 tract-level explanatory variables, which were centred and standardized, ρ m is a vector of associated effect-size parameters, and γ is an ‘intercept’ parameter. We built the main model based on the Deviance Information Criterion (DIC [52] ), on the posterior distribution of the effect-size parameters ( β n in equation (1) and ρ m in equation (3)), and on knowledge of the biological system studied. We first assessed the predictive power of each explanatory variable ( Supplementary Table S1 ) based on the DIC and on the posterior distributions of β n and ρ m . Next, we fitted a multiple model containing the retained explanatory variables. Finally, we simplified this multiple model by excluding and again including earlier excluded variables in a stepwise procedure. Parameter estimates for the final main model for each ecosystem service are presented in Fig. 4 and in Supplementary Table S3 . For some ecosystem services, there were a few models with similar DIC (difference in DIC<2). However, the relationships between the response variables and (i) tree species richness, and (ii) the tree species biomasses differed only marginally between these models. For a description of parameters, symbols and prior distributions, see Supplementary Table S4 . We assumed uninformative prior distributions for all parameters. The models were fitted using the softwares OpenBUGS 2.1 (ref. 53 ). For the models aimed at investigating the pairwise relationships between services, we excluded all plots with missing data. Moreover, bilberry production was also arcsine transformed when used as an explanatory variable. Below follows a detailed description of our response and explanatory variables. Ecosystem services Tree biomass production was estimated as the yearly change in tree biomass (kg m −2 year −1 ), calculated over a period of 5 years, and for all tree individuals higher than 1.3 m. For plots visited in the years 1999–2002, the baseline for biomass production was thus the years 1994–1997. Biomass was calculated with biomass functions [54] , [55] and was the sum of the biomass from the stem, twigs and branches, the stump and roots. For deciduous tree species, there is only a function for Betula spp., and this function was thus applied for all other deciduous tree species. The function for Pinus sylvestris was applied for Larix decidua and Pinus contorta. Even though this creates a slight tree species bias, it has minor effects on our production estimates, as we compared the biomass of the trees at two points in time. Sample size for tree production was 4,335 plots, and due to fallen trees, observed values could be negative (as was the case in 5 plots). Soil carbon storage was measured as the amount of carbon (g m −2 ) in the topsoil, which consisted of either purely organic horizons, for example, mor layers (63%) or peat layers (21%), or less frequently of minerogenic A-horizons (16%). This is the part of the soil most affected by the current above-ground biota. To compensate for the conceptual difference in topsoil types, mean soil carbon stocks were set equal for purely organic soils (measured in the whole organic horizon down to a maximum depth of 30 cm) and minerogenic topsoils (measured in the top 10-cm horizon). The soil fraction <2 mm was analysed. Soil sampling was carried out on around 50% of the inventory plots, totalling 1,953 plots. Data were log transformed. Bilberry production was measured as the percentage of each plot covered by bilberry, Vaccinium myrtillus . The cover of V. myrtillus is strongly correlated to annual production, and bilberry is one of the economically most important wild berry species in Northern Europe [28] . Bilberry sampling was carried out on around 50% of the inventory plots, totalling 2,127 plots. Data were converted to proportions and arcsine transformed, after correcting for the area where berries could not grow, for example, the area of stems and boulders. Game production potential was calculated as the percentage cover of each plot that was covered by any of the 15 plant species important for large herbivorous mammals, for example, moose ( Alces alces ) and roe deer ( Capreolus capreolus ), see Supplementary Table S5 and ref. 56 . The cover of these field layer species was measured in the same way as the bilberry cover. Not all plants are equally preferred, however. Based on known preferences and nutritional values [57] , we therefore weighted the least and most important plant species by 0.66 and 1, respectively ( Supplementary Table S5 ). As the herbivores also browse on coppice, we included the cover of preferred species in this layer ( Supplementary Table S5 ). Field layer and coppice were summed to yield a measure of total food for herbivores, which could amount to more than 100% because of multiple vegetation layers. Game production is the basis for both recreational hunting and meat, and was estimated to a value of US$ 460 million in Sweden as of 2006 (ref. 58 ). Sample size was 2,127 plots and data were log transformed after adding a constant of 0.01. Understory plant species richness: The Swedish National Forest Inventory includes about 270 ground vegetation species, and of these, we selected those with forest as main habitat, in total 141 species ( Supplementary Table S6 ). We modelled the proportion of the richness of these species in each plot in relation to the regional species richness of the same species, estimated as all of the 141 species occurring within a 600 × 600 km window centred on each plot. The regional species pool thus captured the change in species composition with latitude (as the longitudinal distance in the sampling region never exceeds 600 km). We found that the median number of plant species in the regional pool reached an asymptote at a distance of ∼ 300 km from each plot, meaning that further increasing the area of the regional species pool did not, on average, incorporate more species. Sample size was 4,327 plots. We modelled the probability of dead wood occurrence using data on presence/absence of dead wood in each plot (minimum diameter for dead wood pieces to be counted equals 40 mm). We chose this variable, as the abundance of dead wood showed a highly skewed distribution in which small fragments were common and a few plots had very high abundances. Sample size was 4,335 plots. Dead wood is the essential habitat for many organisms: more than 50% of the red-listed forest species in Sweden depend on dead wood [59] . The six ecosystem services included in our analyses are a subset of all possible services that forests provide. The results and conclusions should be viewed with this in mind. Explanatory variables Temperature is defined as the total accumulated average daily temperature (in °C) over 5 °C during the vegetation period. Humidity is measured as the difference in mm between the addition of water via precipitation and the loss of water due to transpiration and evaporation during the vegetation period. For nitrogen deposition, spatially distributed N deposition data in kg N ha −1 year −1 (wet and dry) were downloaded from the Swedish Meteorological and Hydrological Institute website. As temperature, humidity and nitrogen deposition are ‘modelled’ variables, their resolution is not at the scale of local plots, and were thus modelled at the scale of tracts. pH of the topsoil was measured in water suspension. The ratio of total carbon to total nitrogen is the ratio (C:N) in the topsoil. Soil moisture was originally measured on a categorical scale of 1 (driest) to 5 (wettest). These categories correspond to a continuous scale of % volumetric soil water contents ranging from 0.15 to 0.35 (ref. 60 ). Peat was modelled as peat (1) or non-peat (0) soil. The biomass of the six most abundant or regionally important (‘focal’) tree species in Sweden were included. These were: Norway spruce ( Picea abies ), Scots pine ( Pinus sylvestris ), birch ( Betula spp. ; B. pendula and B. pubescens ), oak ( Quercus robur ), aspen ( Populus tremula ) and beech ( Fagus sylvatica ), measured in kg m −2 . Tree species richness was our estimate of tree species diversity. It was calculated as the observed presence of 20 species in each plot, and ranged from 1 to 10. The tree species included our six focal species together with Acer platanoides , Acer pseudoplatanus , Alnus glutinosa , Alnus incana , Carpinus betulus , Fraxinus excelsior , Larix decidua , Pinus contorta , Prunus avium , Salix caprea , Sorbus aucuparia , Sorbus intermedia , Tilia cordata and Ulmus glabra . We chose species richness as our diversity estimate because it is a simple and intuitive measure. Species richness estimates are relatively easy to obtain and relate to the ability to manage ecosystems under limited information about species’ relative distributions and traits. Forest stand age was estimated in each plot as the basal area weighted mean age from at least three trees. How to cite this article: Gamfeldt, L. et al . Higher levels of multiple ecosystem services are found in forests with more tree species. Nat. Commun. 4:1340 doi: 10.1038/ncomms2328 (2013).